Competition between spontaneous symmetry breaking and single-particle gaps in trilayer graphene Many physical phenomena can be understood by single-particle physics; that is, treating particles as non-interacting entities. When this fails, many-body interactions lead to spontaneous symmetry breaking and phenomena such as fundamental particles’ mass generation, superconductivity and magnetism. Competition between single-particle and many-body physics leads to rich phase diagrams. Here we show that rhombohedral-stacked trilayer graphene offers an exciting platform for studying such interplay, in which we observe a giant intrinsic gap ~ 42 meV that can be partially suppressed by an interlayer potential, a parallel magnetic field or a critical temperature ~36 K. Among the proposed correlated phases with spatial uniformity, our results are most consistent with a layer antiferromagnetic state with broken time reversal symmetry. These results reflect the interplay between externally induced and spontaneous symmetry breaking whose relative strengths are tunable by external fields, and provide insight into other low-dimensional systems. In the single-particle picture, rhombohedral trilayer graphene (r-TLG) hosts chiral charge carriers with Berry’s phase 3 π , and an energy-momentum dispersions ε(k) ~ k 3 , thus they are gapless semiconductors ( Fig. 1a inset) [1] , [2] , [3] , [4] , [5] , [6] , [7] . An energy gap can be generated via two different mechanisms, in the single-particle picture, on applying a potential difference U ⊥ between the outmost layers, the band structure adopts a gap that scales with U ⊥ (refs 1 , 2 , 3 , 4 , 5 , 6 , 7 ). Alternatively, close to the charge neutrality point (CNP), the diverging density of states leads to strong electronic interactions, and the gapless semiconductor is expected to give way to phases with spontaneous broken symmetries; in particular, gapped phases such as layer antiferromagnetic (LAF) and quantum anomalous Hall states with broken time reversal symmetry are expected to be favoured [8] , [9] , [10] , [11] , [12] , [13] . Such symmetry-broken states are in direct competition with the U ⊥ -induced single-particle gap, giving rise to a rich phase diagram. 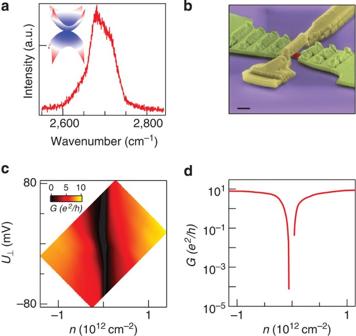Figure 1: Raman spectroscopy, SEM image and transport data of ABC trilayer device. (a) Raman spectroscopy of r-TLG sheet. Inset: energy-momentum dispersion of r-TLG. (b) SEM image of a dual-gated suspended TLG device. Scale bar, 1 μm. (c)G(U⊥, n)in units ofe2/h. (d)G(n)atU⊥=0. Note the logarithmic scale ofG. Figure 1: Raman spectroscopy, SEM image and transport data of ABC trilayer device. ( a ) Raman spectroscopy of r-TLG sheet. Inset: energy-momentum dispersion of r-TLG. ( b ) SEM image of a dual-gated suspended TLG device. Scale bar, 1 μm. ( c ) G(U ⊥ , n) in units of e 2 /h . ( d ) G(n) at U ⊥ =0. Note the logarithmic scale of G . Full size image The rich phase diagram in both zero and finite magnetic field B in r-TLG, lent by the competition between single-particle physics and spontaneous symmetry breaking, has not been explored to date, as most devices previously studied are singly gated and do not allow independent control of both the charge density n and the single-particle term U ⊥ (refs 14 , 15 , 16 , though a gap of ~6 meV was observed in suspended r-TLG [14] ). Here we fabricate dual-gated suspended [17] , [18] , [19] r-TLG devices [20] , where U ⊥ and n can be independently tuned. Device mobility ranges from 20,000 to 90,000 cm 2 V −1 s −1 . Using low temperature transport measurements, we show that, in the absence of external fields, r-TLG at the CNP is an intrinsic insulator, with an energy gap of 42 meV; the critical temperature for transition into this insulating regime is T c ~36 K. This energy gap is partially suppressed by U ⊥ or a parallel magnetic field. Among the spatially uniform correlated phases that have been proposed theoretically [8] , [9] , [10] , [11] , [12] , [13] , our experimental results are most consistent with the presence of a layer antiferromagnet in charge-neutral r-TLG, which is expected to transition into a layer polarized state and a canted ferromagnetic state on the application of external electric and magnetic fields, respectively. Gapped insulating state at the CNP r-TLG sheets on Si/SiO 2 are identified by Raman spectroscopy [21] , [22] ( Fig. 1a ), suspended dual-gated devices ( Fig. 1b ) with mobility as high as 90,000 cm 2 V −1 s −1 are measured in He-3 refrigerators. All measurements are taken at T =260 mK, unless otherwise specified. At low temperatures and B =0, r-TLG devices become insulating in the vicinity of the CNP. In Fig. 1c , the two-terminal differential conductance G=dI/dV from device 1 is plotted as n and U ⊥ . At U ⊥ =0, as n approaches the CNP, G(n) decreases by more than five orders of magnitude to <10 −4 e 2 /h , where e is electron charge and h is Planck’s constant ( Fig. 1d ). This insulating state at the CNP is extremely robust, as it persists for the entire gate ranges up to the highest applied U ⊥ (~65 mV). Transport spectroscopy [17] , [19] at n=U ⊥ =0 reveals intriguing features: at small source-drain bias V , the device stays insulating, but as V increases±42 mV, G rises by more than six orders of magnitude to extremely sharp peaks, then decreases to ~15 e 2 /h for larger V ( Fig. 2a ). Such a G(V) curve strongly resembles the density of state of a gapped phase, suggesting the presence of an energy gap Δ ~42 meV at n=U ⊥ = B =0. With increasing charge density n , the gap diminishes and eventually disappears entirely ( Fig. 2b ). At n =3 × 10 11 cm −2 , G(V) is flat, indicating that r-TLG becomes gapless at high density. 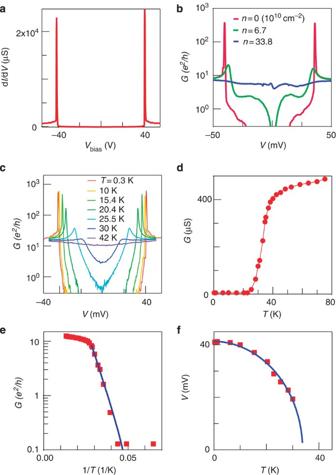Figure 2: Transport data atB⊥=0 (a,b: Device 1;c–f: Device 2). (a)G(V)atU⊥=n=0. (b)G(V)atU⊥=0 and differentn. (c)Gmin(V)atU⊥=n=0 and different temperatures. (d)GminatV=0 versusT. (e)Gminversus 1/Tin Arrhenius scale. The blue line is a fit to the equationfor 30 K<T<40 K. (f) MeasuredΔas a function ofT. The solid line is a fit to equation (1). Figure 2: Transport data at B ⊥ =0 ( a , b : Device 1; c – f : Device 2). ( a ) G(V) at U ⊥ = n= 0. ( b ) G(V) at U ⊥ =0 and different n . ( c ) G min (V) at U ⊥ = n= 0 and different temperatures. ( d ) G min at V= 0 versus T . ( e ) G min versus 1/ T in Arrhenius scale. The blue line is a fit to the equation for 30 K< T <40 K. ( f ) Measured Δ as a function of T . The solid line is a fit to equation (1). Full size image The gapped, insulating state near the CNP in the absence of external fields is unexpected from tight-binding calculations, but instead suggests a phase arising from electronic interactions with spontaneous broken symmetries [23] . The magnitude of the gap, ~42 meV, is exceedingly large for an interaction-induced state. It is more than an order of magnitude larger than that found in BLG [17] , [24] , reflecting the divergent nature of the density of states and strong electronic interactions in r-TLG at the CNP. It also a factor of seven larger than that previously observed in singly gated devices [14] , likely due to improved device geometry and quality. Temperature dependence of the gapped state To further establish the magnitude of the gap, we examine temperature dependence of G(V) at n=U ⊥ =0 ( Fig. 2c ). Figure 2d plots minimum conductance G min = G(V=0) as a function of T. At high temperatures T >40 K, the device is conductive, G min ~15 e 2 /h with a small linear T -dependence. The G(V) curves are approximately constant, similar to that of a conventional resistor. However, when T <~40 K, G min drops precipitously and becomes insulating for T< 30 K, and G(V) curves develop prominent peaks at finite V . In the transition region 30< T <40 K, the G min (T) curve is well-described by the thermal activation equation, ( Fig. 2e ), where k B is the Boltzmann’s constant and Δ ~43 meV is obtained as a fitting parameter. This is in excellent agreement with the value of Δ obtained from G(V) curves at T =300 mK, thus confirming the presence of an insulating state with ~42±1 meV gap. Using G(V) curves, we can also directly measure the evolution of Δ (taken as half of the peak-to-peak separation in V ) as a function of T . As shown in Fig. 2f , Δ is almost constant for T< 10 K, but drops precipitously for T >30 K. This behaviour is a characteristic of order parameters during phase transitions in mean field theories. Thus, we fit Δ(T) to the function [25] where T c is the critical temperature. Equation (1) reduces to the usual mean –field functional form for T/T c sufficiently close to 1, and the second term is inserted to capture the vanishingly small dependence on T as T →0. Excellent agreement with data is obtained, yielding A= 2.0, B =−1.0 and T c =34 K. The energy scale of the gap, Δ(0)/k B =500 K, which is much larger than that associated with the critical temperature, signifies that this insulating state observed at the CNP is a correlated phase. E and B || field dependence of the gapped state To elucidate the nature of this correlated phase, we examine how it is modified in the presence of an external field that selectively breaks one of the degeneracies. For instance, application of U ⊥ breaks the inversion (which-layer) symmetry, and, in the single-particle picture, gives rise to a proportionally scaled energy gap. 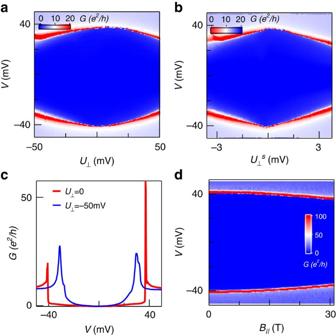Figure 3: Transport data atn=0 and finiteU⊥andB||. (a,b)G(V,U⊥) andin units ofe2/hfrom Device 1. (c) Line tracesG(V)atU⊥=0 andU⊥=−50 mV. (d)G(V,B||) in units ofe2/hfrom Device 2. Figure 3a displays G as a function of V and U ⊥ at n =0. As U ⊥ is the externally imposed potential bias, it will be heavily screened due to r-TLG’s large density of states near the CNP [26] , [27] , [28] . Thus, we expect the screened interlayer potential bias . Using a simplified two-band Hamiltonian for r-TLG and assuming that the dielectric constant of r-TLG is 1, we self-consistently calculate for given values of n and U ⊥ (see Supplementary Note 1 for detail): Figure 3: Transport data at n =0 and finite U ⊥ and B || . ( a , b ) G(V , U ⊥ ) and in units of e 2 /h from Device 1. ( c ) Line traces G(V) at U ⊥ =0 and U ⊥ =−50 mV. ( d ) G(V , B || ) in units of e 2 /h from Device 2. Full size image where , γ 1 is the interlayer hopping parameter, v the Fermi velocity of charges in monolayer graphene, d =0.67 nm is the spacing between outmost layers (for derivation of equation (2), see Supplementary Note 1 ). The screening-corrected data are shown in Fig. 3b .The sharp peaks in G(V) , that is, the gap edges, appear as red curves that separate the insulating (dark blue) and conductive (light blue) regions in Fig. 3a,b . Δ decreases symmetrically and linearly with applied of either polarity, to ~30 meV at | U ⊥ |=50 mV or ( Fig. 3b ), though not yet completely closed at the largest applied | U ⊥ |. (In other devices with lower mobility, we also observe that the device conductance increases from <0.1 e 2 /h with increasing | U ⊥ |, exceeding 1.5 e 2 /h at | U ⊥ |=85 mV, as shown in Supplementary Fig. 2 ). In contrast, an in-plane magnetic field B || couples to the spin but not orbital degrees of freedom and raises the Zeeman energy. Figure 3d plots G(V , B || ) for B || =0 to 31T. Δ stays almost constant for B || <10T, but decreases to 35 mV at B || =31T. Thus, addition of Zeeman energy suppresses the gapped phase, suggesting that the phase has spin-ordering, but no net magnetic moment. To summarize our experimental findings, we observe an insulating state in r-TLG at n= U ⊥ = B =0, with an energy gap Δ(T=0) ~42 meV. This gap can be suppressed by increasing charge density n , a critical temperature T c ~34 K, by an interlayer potential U ⊥ of either polarity and by an in-plane magnetic field. Among the spatially uniform correlated phases in r-TLG discussed in the literature [8] , [9] , [10] , [11] , [12] , [13] , only LAF, in which the top and bottom layers have equal number of electrons with opposite spin polarization, is consistent with our experimental observations. For instance, the presence of an energy gap eliminates the mirror-breaking, inversion breaking, interlayer current density wave or layer polarization density wave states [12] , and the zero conductance eliminates the superconductor, quantum spin Hall and quantum anomalous Hall states that host finite (or even infinite) conductance. Furthermore, the symmetrical suppression of the gap by U ⊥ of either polarity suggests that charges in the insulating state are layer-balanced, as the device would otherwise exhibit opposite dependence on U ⊥ of opposite polarities. This excludes all layer-polarized states, including the quantum valley Hall and layer polarization density wave states, and any single-particle state that arises from inadvertent doping of one of the surface layers. Thus, based on the above experimental observations, we identify LAF with broken time reversal and spin rotation symmetries as the most likely candidate among the proposed ground states in r-TLG. Theoretically, an LAF ground state can be justified by the following considerations. The strong screening due to the large density of states in r-TLG leads to very short range Coulomb repulsions among electrons (see Supplementary Note 3 ). For such local interactions, the most likely symmetry-broken states are the LAF and nematic phases, and the gapless and conductive nematic phase is incompatible with our observation of a gapped insulator, leaving LAF as the only viable alternative. Moreover, mean field arguments that generally favour the LAF phase should be more robust in r-TLG than that in bilayer graphene, due to the divergent density of states and stronger electrons near the CNP that suppresses fluctuations. Finally, recent works [29] , [30] report formation of magnetic moments in graphene that results from interactions among the π-electrons of graphene in the presence of hydrogen and fluorine atoms and vacancies, thus it is not unreasonable to expect emergent magnetism arising from strong electronic interactions in r-TLG. Within the mean-field framework, a simple estimate of the LAF gap yields (see Supplementary Note 4 ) where γ 0 ≈2.7 eV, γ 1 ≈0.4 eV are tight binding parameters, c ≈2.8, and U is the Hubbard onsite interaction. Using these parameters, and substituting the experimentally obtained value Δ =42 meV, we obtain U ~13 eV, not too different from theoretically predicated values of 5–10 eV (refs 31 , 32 , 33 ). Alternatively, the gap can be further enhanced by exchange processes associated with the long-range part of the interaction [31] . A possible phase diagram for charge neutral r-TLG that is consistent with our experimental results, together with schematics for electron configurations, is summarized in Fig. 4 . In the absence of external fields, a charge neutral r-TLG is an LAF with broken time reversal and spin rotation symmetries. Increasing U ⊥ of either polarity pushes electrons to one of the surface layers and suppresses the gap. For sufficiently large | U ⊥ |, all charges reside in either the top or bottom layer, giving rise to a quantum valley Hall (QVH) insulator with broken inversion symmetry. We note that the different broken symmetries of the QVH and LAF states preclude a continuous phase transition between them [5] , [34] , [35] . In contrast, as B || increases from 0, the competition between the Zeeman and the exchange energies tilts the electron spins, and r-TLG crosses over to the CAF phase. For very large B || , we expect that the electrons eventually form a ferromagnet (F); in the quantum Hall regime, this ferromagnet is analogous to a quantum spin Hall state, with counter-propagating edge states and conductance ~6 e 2 /h (ref. 36 ). 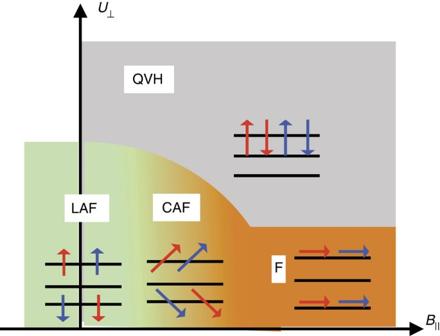Figure 4: Possible phase diagram and schematics of electronic configurations for r-TLG. The blue and red arrows indicate charges from K and K′ valleys, respectively. (CAF, canted antiferromagnet; F, ferromagnet; LAF, layer antiferromagnet; QVH, quantum valley Hall). Figure 4: Possible phase diagram and schematics of electronic configurations for r-TLG. The blue and red arrows indicate charges from K and K′ valleys, respectively. (CAF, canted antiferromagnet; F, ferromagnet; LAF, layer antiferromagnet; QVH, quantum valley Hall). Full size image Sample preparation Trilayer graphene sheets are mechanically exfoliated onto 300 nm SiO 2 wafer layer grown over degenerately doped Si. ABC or rhomborohedral stacked trilayer (r-TLG) sheets are selected by colour contrast in optical microscope [37] and Raman spectroscopy [21] , [22] , coupled to electrodes and top gates using multi-level lithography [38] , [39] , and etched in HF to partially remove the SiO 2 layer. All devices have source-drain separation ~1.1 μm and width ~1.1–1.4 μm. Characterization of devices Most as-fabricated devices have low mobility, and current annealing is performed at 4 K to improve sample quality [40] , [41] . Typically the optimal annealing results are achieved when current starts to saturate, at ~0.3~0.4 mA μm −1 layer −1 . After annealing, device mobility is as high as 90,000 cm 2 V −1 s −1 . Supplementary Figure 1 displays the conductance G of a typical r-TLG device as a function of back gate voltage V bg before and after annealing. The field-effect mobility of this device after annealing is ~50,000 cm 2 V −1 s −1 , with a minimum conductivity ~0. The devices are measured in helium-3 refrigerators using standard lock-in techniques. Calculation of charge density and interlayer potential For a given device, the induced charge density n and interlayer potential U ⊥ are calculated from the back gate and top gate voltages, n =( C bg V bg + C tg V tg )/ e and U ⊥ =( C bg V bg − C tg V tg ) d /2 ε 0 . Here e is electron charge, ε 0 the permittivity of vacuum, d =0.67 nm is the distance between the top and bottom layers, V bg and V tg are the voltage applied to back gate and top gate, respectively, and C bg ( C tg ) is the capacitance per unit area between graphene and back (top) gate. Capacitances are estimated from geometric considerations, as well as from standard Landau level fan diagrams. For typical devices, C bg / e ranges from 3 × 10 10 to 5 × 10 10 cm −2 , and C tg /e from 1 × 10 10 to 7 × 10 10 cm −2 . How to cite this article : Lee, Y. et al . Competition between spontaneous symmetry breaking and single-particle gaps in trilayer graphene. Nat. Commun. 5:5656 doi: 10.1038/ncomms6656 (2014).